Evidence for infragravity wave-tide resonance in deep oceans Ocean tides are the oscillatory motions of seawater forced by the gravitational attraction of the Moon and Sun with periods of a half to a day and wavelengths of the semi-Pacific to Pacific scale. Ocean infragravity (IG) waves are sea-surface gravity waves with periods of several minutes and wavelengths of several dozen kilometres. Here we report the first evidence of the resonance between these two ubiquitous phenomena, mutually very different in period and wavelength, in deep oceans. The evidence comes from long-term, large-scale observations with arrays of broadband ocean-bottom seismometers located at depths of more than 4,000 m in the Pacific Ocean. This observational evidence is substantiated by a theoretical argument that IG waves and the tide can resonantly couple and that such coupling occurs over unexpectedly wide areas of the Pacific Ocean. Through this resonant coupling, some of ocean tidal energy is transferred in deep oceans to IG wave energy. Infragravity (IG) waves are surface waves that are observed in deep [1] and coastal [2] oceans. IG waves are strongest near the shoreline [3] , where they cause harbour oscillations and near-shore processes such as sediment transport [4] . Disturbances due to IG waves make it difficult to interpret long-period seismograms at the ocean bottom [5] , [6] . Forcing of IG waves is believed to be a major source of Earth's background free oscillations (also known as Earth's hum) [7] , [8] , [9] , [10] , [11] , [12] , [13] , [14] . IG waves are mainly generated through nonlinear interactions between high-frequency (period: 20–5 s) wind waves [15] , [16] . There are a few reports on the tidal modulation of IG waves in coastal oceans (water depth: 10–30 m) [17] , [18] , [19] and that on the 1,000-m-deep shelf [6] , where the IG wave energy is reduced at low tide. The suggested mechanisms for tidal modulation emphasize the influence of the tide on the generation or decay of IG waves in shallow seas [19] , [20] . No tidal modulation has been reported for IG waves in open seas or deep oceans. Here we present the first evidence of the resonance between IG waves and the tide in deep oceans, and show that such resonance can occur over wide areas of the Pacific Ocean. Modulation of IG waves by ocean tide We analysed the continuous vertical component records obtained from two broadband ocean-bottom seismometer (BBOBS; sensor: Guralp CMG-3T) arrays: one (1 February 2003–31 January 2004) with 7 stations (FP array), deployed in French Polynesia [21] and the other (1 December 2006–30 November 2007) with 11 stations (PS array), deployed in the northern Philippine Sea [22] . 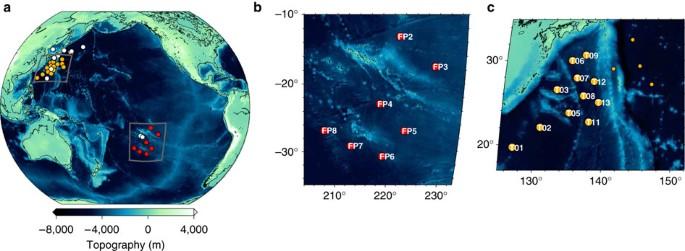Figure 1: Station distribution map. Geographical distributions of the stations in the French Polynesia (FP) array21(close-up inb) and Philippine Sea (PS) array22(close-up inc). These stations are mostly located at depths of 4,000–5,000 m. We analysed the continuous vertical records at 7 FP-array stations (red circles) available between 1 February 2003 and 31 January 2004 and those at 11 PS-array stations (orange circles) available between 1 December 2006 and 30 November 2007. For the PS array, only the results obtained for the seven western stations are shown inFigure 4. The stations of the PS array not considered in the analysis are shown by orange dots. The BBOBS stations not belonging to the FP and PS arrays are shown by white circles ina. Figure 1 shows the geographical distributions of the stations in these two arrays, which are mostly located at depths of 4,000–5,000 m. Details of the observations are provided in the Methods section. 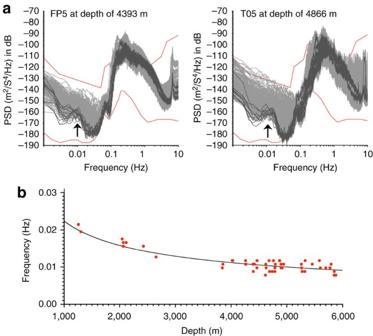Figure 2: Infragravity wave signature on the seafloor noise spectra. (a) Seafloor noise spectra at station FP5 for the period 14 January 2003 and 14 January 2004 and those at T05 for the period 11 November 2006–11 November 2007. Each of the power spectra is calculated using the standard procedure followed in seismology29, for a record-section length of 4,096 s and sampling rate of 100 Hz. The 10 spectral lines with the lowest noise amplitudes in the frequency range 0.02–0.05 Hz are blackened to show the noise spectra typical to quiet days. The spectral peak∼0.01 Hz (indicated by the arrow) represents the disturbance due to infragravity (IG) waves. The two red curves indicate the New Low Noise Model (NLNM) and New High Noise Model (NHNM) of Peterson29. (b) Plot of the peak frequencyf0(in Hz) in the infragravity band against seafloor depthH(in m). Data are obtained from all the BBOBS stations shown inFigure 1. The plots are approximated by the relationf0=(2H)−1/2. This relation is understood ask0H≈1.4, which can be expected if the hydrodynamic filtering of IG waves1is responsible for the peak. Figure 2a shows two examples of seafloor noise spectra, one obtained from the FP array and the other obtained from the PS array. It has been reported that the spectral peak appearing at ∼ 10 mHz is a signature of the seafloor disturbance caused by IG waves [1] , [5] . This interpretation is supported by Figure 2b , which shows that the depth dependence of the peak frequency in the IG band can be attributed to the hydrodynamic filtering of IG waves. 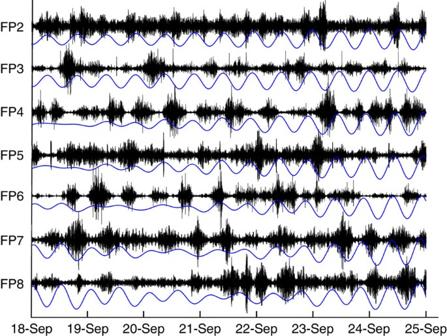Figure 3: Seismograms filtered through the IG-band. Example of the FP array records (18–25 September 2003) bandpass filtered between 4 and 20 mHz. The dominant signal in this band is the seafloor disturbance due to IG waves. The IG wave trains show temporal variations on a semidiurnal to diurnal scale. The theoretical tidal sea level changes are shown below each record25. Figure 3 shows the FP array records that are bandpass-filtered between 4 and 20 mHz; in this frequency range, the signal due to the IG waves is dominant. The IG wave trains show temporal variations on a semidiurnal to diurnal scale; however, visual inspection does not reveal any unique periodicity in time coherent through the array. In order to detect any semidiurnal or diurnal periodicity in the IG wave activity coherent across the stations, we divided the 1-year record obtained from a station into ∼ 30-day (2.8 × 10 6 s)-long segments with an overlap of ∼ 10 days (1.0 × 10 6 s). Each of the 30-day-long segments was bandpass filtered between 4 and 20 mHz to extract the IG signals. The negative IG signals were reversed in sign in order to obtain an absolute-value time series, which was used as a measure of the IG wave activity. The persistency of temporal periodicity among different stations in the same sampling period was examined by normalizing the maximum amplitude of each 30-days long record and by calculating a cross-spectrum Q ij ( f ) between stations i and j (≠ i ). The temporal persistence of the periodicity was examined by constructing cross-spectrograms. The cross-spectrogram for a station pair i and j is a plot of the cross-spectral power | Q ij ( f )| against time. For ease of illustration, we define the stacked cross-spectrogram for the i th station as a stack of the cross-spectrograms obtained for all pairs of the i th station and the other stations in the same seismic array. 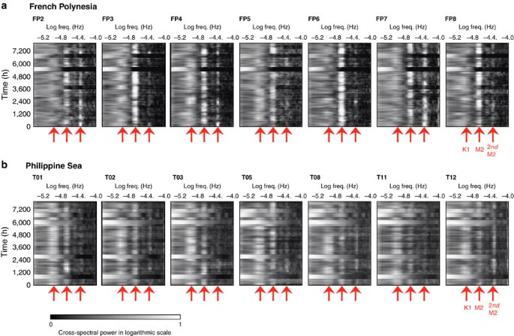Figure 4: Stacked cross-spectrograms. Stacked cross-spectrogram for each of the stations of the (a) FP and (b) PS arrays. The stacked cross-spectrogram for a station is a stack of the cross-spectrograms for all the pairs of that station and the other stations in the same seismic array. Each record is normalized by its maximum amplitude. The arrows along the frequency axis indicate the principal solar tide K1, the principal lunar tide M2and the second harmonic of M2, respectively, in the order of increasing frequency. Figure 4 shows the stacked cross-spectrograms so defined. The frequency f K 1 (period: 23.93 h) of the principal solar tide K 1 , frequency 2 f M 2 (period: 12.42 h) of the principal lunar tide M 2 , and its double frequency 2 f M 2 are indicated by arrows along the frequency axis of each stacked cross-spectrogram. Note that the intervals between f K 1 and f M 2 and between f M 2 and 2 f M 2 are not equal to each other. The spectral peaks at these three frequencies can be recognized in the spectrograms for almost all time periods and across all the stations. The M 2 signal is much stronger in the FP spectrograms than in the PS spectrograms, whereas the intensity of the K 1 signal is almost the same in the FP and PS spectrograms. The second harmonic of the M 2 signal is considerably weaker than the first harmonic in both the FP and PS spectrograms. Figure 1: Station distribution map. Geographical distributions of the stations in the French Polynesia (FP) array [21] (close-up in b ) and Philippine Sea (PS) array [22] (close-up in c ). These stations are mostly located at depths of 4,000–5,000 m. We analysed the continuous vertical records at 7 FP-array stations (red circles) available between 1 February 2003 and 31 January 2004 and those at 11 PS-array stations (orange circles) available between 1 December 2006 and 30 November 2007. For the PS array, only the results obtained for the seven western stations are shown in Figure 4 . The stations of the PS array not considered in the analysis are shown by orange dots. The BBOBS stations not belonging to the FP and PS arrays are shown by white circles in a . Full size image Figure 2: Infragravity wave signature on the seafloor noise spectra. ( a ) Seafloor noise spectra at station FP5 for the period 14 January 2003 and 14 January 2004 and those at T05 for the period 11 November 2006–11 November 2007. Each of the power spectra is calculated using the standard procedure followed in seismology [29] , for a record-section length of 4,096 s and sampling rate of 100 Hz. The 10 spectral lines with the lowest noise amplitudes in the frequency range 0.02–0.05 Hz are blackened to show the noise spectra typical to quiet days. The spectral peak ∼ 0.01 Hz (indicated by the arrow) represents the disturbance due to infragravity (IG) waves. The two red curves indicate the New Low Noise Model (NLNM) and New High Noise Model (NHNM) of Peterson [29] . ( b ) Plot of the peak frequency f 0 (in Hz) in the infragravity band against seafloor depth H (in m). Data are obtained from all the BBOBS stations shown in Figure 1 . The plots are approximated by the relation f 0 =(2 H ) −1/2 . This relation is understood as k 0 H ≈1.4, which can be expected if the hydrodynamic filtering of IG waves [1] is responsible for the peak. Full size image Figure 3: Seismograms filtered through the IG-band. Example of the FP array records (18–25 September 2003) bandpass filtered between 4 and 20 mHz. The dominant signal in this band is the seafloor disturbance due to IG waves. The IG wave trains show temporal variations on a semidiurnal to diurnal scale. The theoretical tidal sea level changes are shown below each record [25] . Full size image Figure 4: Stacked cross-spectrograms. Stacked cross-spectrogram for each of the stations of the ( a ) FP and ( b ) PS arrays. The stacked cross-spectrogram for a station is a stack of the cross-spectrograms for all the pairs of that station and the other stations in the same seismic array. Each record is normalized by its maximum amplitude. The arrows along the frequency axis indicate the principal solar tide K 1 , the principal lunar tide M 2 and the second harmonic of M 2 , respectively, in the order of increasing frequency. Full size image A theory of the resonance between IG waves and the ocean tide A theory was developed for the coupling of IG waves with the tide in a long-wave approximation. Details of this theory are provided in the Methods section. The wave field is assumed to be a random, homogeneous superposition of free IG waves of the form where is the horizontal wavenumber vector and (ref. 23 ). This assumption is justified by observations made in the deep ocean [1] . The angular frequency ω is related to k as , where c is the frequency-independent propagation speed; g , the gravitational acceleration; and H , the water depth. The tidal motion in the local coordinates can be expressed as so that the co-phase line of the ocean tide with an angular frequency Ω moves in the direction given by the wavenumber vector and with a speed defined by C ≡Ω/ K . The fluid-dynamic equation of motion including the advection term has a solution of the form showing the tide-modulated IG waves, where the amplification factor R is proportional to In a homogenous random wave field, there is always a wavenumber vector such that with which R undergoes resonant divergence, if Comparison of the observations and theory We calculated R for the Pacific Ocean by using the global bathymetry model of ETOPO2 [24] and an ocean tidal model developed by Matsumoto et al . [25] We set the ω value to the peak frequency in the IG wave band of the seafloor noise at each observational site, as shown by the arrow in Figure 2a . 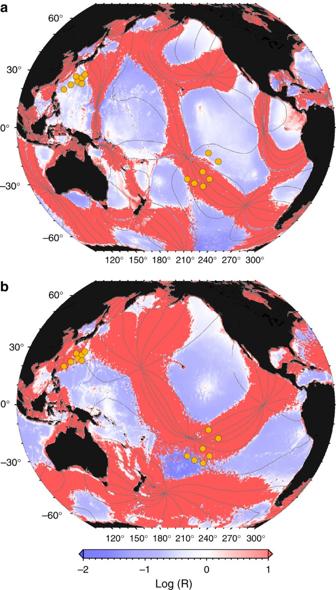Figure 5: Maps of amplification factorRfor infragravity waves–ocean tides coupling. Ris a measure of how large the coupled-wave amplitude is relative to the amplitude of the undisturbed wave. The area that is practically in a resonant state is coloured in red. The whitish area may be understood to be in a near-resonant state. The tidal co-phase lines are contoured. White dots indicate the amphidromic points. Map (a) for the M2tide and (b) for the K1tide. Figure 5a,b show the maps of R for the M 2 and K 1 tides, respectively. The area coloured in red is essentially in resonant state, as defined by inequality (1), which may be approximated as c ≥ C . For a 4,000-m ocean depth, c ≈200 m s −1 , whereas the tidal co-phase line at latitude ϑ is expected to move westward with a speed C ≈450×cos ϑ m s −1 , if a laterally uniform ocean covers a laterally uniform Earth. This implies that for a 4,000-m-deep uniform ocean, resonance is expected only at high latitudes ( ϑ ≳ 65°). Figure 5 demonstrates how different the resonance in the real ocean is from that in the uniform model ocean. In Figure 5 , the white area is understood to be in a near-resonance state, where the precise value of R is not calculable according to our first-order perturbation theory. We can see that unexpectedly wide areas of the Pacific Ocean are in the resonant or near-resonant state. A major part of the FP array is within the resonant area for the M 2 tide, whereas a major part of the PS array is outside the resonant area; this would be the reason for the M 2 signal being stronger in the FP array than in the PS array ( Fig. 4 ). On the other hand, a major part of either array is within the resonant area for the K 1 tide, explaining that the K 1 signal intensities in the FP and PS arrays are not very different ( Fig. 4 ). Figure 5: Maps of amplification factor R for infragravity waves–ocean tides coupling. R is a measure of how large the coupled-wave amplitude is relative to the amplitude of the undisturbed wave. The area that is practically in a resonant state is coloured in red. The whitish area may be understood to be in a near-resonant state. The tidal co-phase lines are contoured. White dots indicate the amphidromic points. Map ( a ) for the M 2 tide and ( b ) for the K 1 tide. Full size image Although the above-mentioned observations clearly indicate that IG waves in the deep ocean recorded by the BBOBSs are persistently modulated by tidal disturbances, there is a possibility of these waves being apparently modulated by the tide-related sensitivity change of the instrument. Such a sensitivity change may be caused by tilting of the sensor axis due either to the tidal currents or to the solid Earth tide. Either possibility, however, is unlikely, as will be explained below. 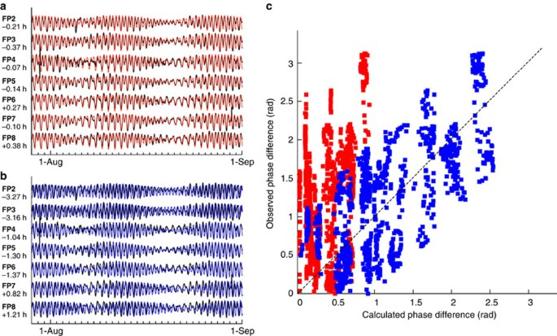Figure 6: Seismograms and comparison of observed and calculated cross-spectral phases. (a,b) Example of the FP array records (31 July–31 August 2003) filtered through the tidal band and corrected for the instrumental response. Comparison is made with (a) the gravity component (or vertical displacement) of the theoretical solid Earth tide25and (b) the sea level change (or horizontal velocity) of the theoretical ocean tide25. The value attached to each paired trace indicates the relative time shift that yields the best waveform match. (c) Plots of theoretical cross-spectral phases for the tilt of the solid Earth tide and for the sea level change of the ocean tide against the observed cross-spectral phase for the IG wave activity at the M2tidal frequency. Plots are made for every station pair in the FP array if the observed cross-spectral power at the M2tidal frequency is >0.95 times the maximum cross-spectral power. A phase in the range 0–2πis reduced to that in the range 0–πby appropriately subtractingπ. If the observed and theoretical cross-spectral phases coincide with each other, the plots should lie on the dotted straight line. Figure 6a,b shows comparisons of the theoretical tides with the tidal-band records of the FP array corrected for the instrumental response. In Figure 6a, the comparison is made for the gravity component (corresponding approximately to the vertical displacement) of the theoretical solid Earth tide [25] . In Figure 6b, the comparison is made for the sea level change (corresponding approximately to the horizontal velocity) of the theoretical ocean tide [25] . The value attached to each pair of the observed and theoretical traces is a lag-time τ to obtain the best waveform match. In Figure 6a , the observed and theoretical traces are in almost in phase ( τ always <0.4 h), indicating that the observed traces are almost π /2 out of phase with the tilt component of the solid tide. In Figure 6b , the observed and theoretical traces are not in phase, where τ increases systematically (from −3.3 to +1.2 h) as we move southwestward through the array (from FP2 to FP8, Fig. 1 ). Clearly, the vertical records in the tidal band are dominated by the gravity signal due to the solid Earth tide. There is no indication for the vertical records being affected by tilting of the instrument due either to the seafloor tilt or to the tidal current at the BBOBS site. The observed tidal modulation of IG waves should be an actual process occurring in the ocean, rather than an apparent phenomenon caused by the instrumental tilting. Figure 6: Seismograms and comparison of observed and calculated cross-spectral phases. ( a , b ) Example of the FP array records (31 July–31 August 2003) filtered through the tidal band and corrected for the instrumental response. Comparison is made with ( a ) the gravity component (or vertical displacement) of the theoretical solid Earth tide [25] and ( b ) the sea level change (or horizontal velocity) of the theoretical ocean tide [25] . The value attached to each paired trace indicates the relative time shift that yields the best waveform match. ( c ) Plots of theoretical cross-spectral phases for the tilt of the solid Earth tide and for the sea level change of the ocean tide against the observed cross-spectral phase for the IG wave activity at the M 2 tidal frequency. Plots are made for every station pair in the FP array if the observed cross-spectral power at the M 2 tidal frequency is >0.95 times the maximum cross-spectral power. A phase in the range 0–2 π is reduced to that in the range 0– π by appropriately subtracting π . If the observed and theoretical cross-spectral phases coincide with each other, the plots should lie on the dotted straight line. Full size image This is further confirmed in Figure 6c , which compares the phase of the observed cross-spectrum with and in the same sampling period. Here, and are the cross-spectral phases of the tilt component of the theoretical solid Earth tide and the sea surface elevation of the theoretical ocean tide [25] , respectively. The cross-correlation function of the observed time series takes only positive values, whereas the cross-correlation functions of the theoretical tides take both positive and negative values. To account for this difference, a phase in the range 0–2 π is reduced to that in the range 0– π . In Figure 6c , the values of and are plotted against for the FP array for the cases where is very large (more than 0.95 times the maximum of over the frequency range shown in Fig. 4 ). It is apparent that is in better agreement with than with The agreement of with and the absence of ocean tide signals on the records in the tidal band ( Fig. 6c ) indicate that tidal modulation occurs by coupling between IG waves and the ocean tide in the deep ocean, and not by tide-induced tilting of the sensor axis. If this is the case, the propagation of IG waves may not be perfectly isotropic [1] , but preferentially parallel to the direction of the co-phase lines. This hypothesis can be tested by carrying out long-term, dense-array observations of the pressure changes at the sea bottom. We have shown that free IG waves in the deep ocean are amplified by the resonance with ocean tides and that such resonance can occur over wide areas of the Pacific Ocean. This implies that ocean tides dissipate a certain amount of energy through resonant coupling with IG waves. Our findings suggest the existence of a possible driving force for IG waves in deep oceans and a possible dissipation mechanism of ocean tidal energy in deep oceans [26] , [27] . A theory of the resonance between IG waves and the ocean tide Herein, we present a theory of the resonant coupling between IG waves and the ocean tide. In a long-wave approximation, the two-dimensional equation of motion and the equation for conservation of mass are written as where is the horizontal velocity vector; ξ , the sea surface elevation; g , the gravitational acceleration; φ , the tidal potential; and H , the water depth [28] . When H =const and ζ ≪ H , To obtain the first-order solution, we ignore the nonlinear advection term in (2): Under the assumption that the wave field is random and homogeneous [23] , the free-wave solution can be given as where and The free-wave (IG wave) propagates in the direction defined by the wavenumber vector with a frequency-independent speed c . We express the free-wave-induced sea surface elevation as Substituting this expression in the linearized second equation in (1), we obtain Without taking into account the detailed form of the tidal potential, we assume that the tidal response can be locally expressed in terms of the horizontal velocity as follows: so that the co-phase line of the tide moves in the direction defined by the wavenumber vector with a speed defined by The height variation associated with (8) is with The first-order solution is then written as In a more general case, we assume that the fluid velocity can be expanded in a perturbation series where the first-order term is given by (12) [23] . To determine we must make allowance for the nonlinear term. The solution can be obtained by solving the following equation: When (12) is introduced on the right-hand side of (13) and only the interaction terms between free waves and the tide are retained, (13) reduces to The particular solution of (14) is given by where and Condition for the resonance between IG waves and the ocean tide : If there is a wavenumber vector , such that in a homogeneous random wave field. With such a value, either or becomes infinite in (15), and hence, the IG wave resonates with the tide. The resonance area in the Pacific Ocean, as defined by (17), is shown for the M 2 tide in Figure 5a and for the K 1 mode in Figure 5b . No resonance occurs if where the sine–sine modulation term dominates the cosine–cosine term in (15). The amplitude of the IG wave becomes maximum when the wavenumber vectors and are in the same direction, so that where Thus, in the case of (19), the interaction of an IG wave packet with the tide results in a tide-modulated IG wave packet whose amplitude is R times that of the original wave packet. This amplification factor R may be rewritten as follows, by using (5) and (11): For the non-resonant area in the Pacific Ocean, as defined by (19), R is plotted for the M 2 tide in Figure 5a and for the K 1 mode in Figure 5b . Note that the plane-wave approximations, as in (8) and (10), may not be valid near the amphidromic point around which the tidal system rotates [28] . The behaviour near the amphidromic point is beyond the scope of our theory. Broadband seismic observation at sea bottoms The BBOBS system has been developed by the Earthquake Research Institute of the University of Tokyo since the 1990s. A BBOBS unit is a self-pop-up type, designed to rise from the seafloor after receipt of an acoustic command. The BBOBS with a three-component CMG-3 T broadband sensor (Guralp Systems) senses ground motions at periods from 0.02 to 360 s with a sampling rate of 100 Hz at 24-bit resolution. All of the seismic instrument components, including the sensor, data logger, transponder and batteries, are packed into a 65-cm diameter titanium alloy pressure housing, which allows for a maximum operating depth of 6,000 m. The system runs for as long as 500 days to ensure long-term seismic observations. We have practiced more than 50 long-term BBOBS experiments since 1999, including several array observations at the Pacific Ocean seafloor. The locations of all the BBOBS stations are shown in Figure 1 . How to cite this article: Sugioka, H. et al . Evidence for infragravity wave-tide resonance in deep oceans. Nat. Commun. 1:84 doi: 10.1038/ncomms1083 (2010).